TRPM7 is essential for Mg2+homeostasis in mammals Mg 2+ is the second-most abundant cation in animal cells and is an essential cofactor in numerous enzymatic reactions. The molecular mechanisms controlling Mg 2+ balance in the organism are not well understood. In this study, we report identification of TRPM7, a bifunctional protein containing a protein kinase fused to an ion channel, as a key regulator of whole body Mg 2+ homeostasis in mammals. We generated TRPM7-deficient mice with the deletion of the kinase domain. Homozygous TRPM7 Δ kinase mice demonstrated early embryonic lethality, whereas heterozygous mice were viable, but developed signs of hypomagnesaemia and revealed a defect in intestinal Mg 2+ absorption. Cells derived from heterozygous TRPM7 Δ kinase mice demonstrated reduced TRPM7 currents that had increased sensitivity to the inhibition by Mg 2+ . Embryonic stem cells lacking TRPM7 kinase domain displayed a proliferation arrest phenotype that can be rescued by Mg 2+ supplementation. Our results demonstrate that TRPM7 is essential for the control of cellular and whole body Mg 2+ homeostasis. It was recently suggested [1] that Mg 2+ uptake in mammalian cells is mediated by the channel kinases TRPM7 [2] , [3] and TRPM6 [4] , [5] , which are unusual bifunctional molecules representing the only known vertebrate proteins consisting of an ion channel fused to a protein kinase. Under physiological conditions, TRPM7 passes weak inward current and is permeable to a number of divalent metal cations, including Mg 2+ and Ca 2+ , as well as trace metal ions such as Mn 2+ , Co 2+ and Zn 2+ (refs 3 , 6 ). The current is inhibited by free Mg 2+ or Mg·ATP [3] . The kinase catalytic domain of TRPM7 belongs to the family of atypical protein kinases known as alpha kinases [7] , [8] , [9] . Deficiency of TRPM7 in DT-40 chicken lymphoma cells results in cell cycle arrest; the proliferation of these cells can be rescued by increasing the extracellular magnesium concentration [1] . It was suggested that the channel part of TRPM7 can serve as a major Mg 2+ uptake pathway into the cell, whereas the changes of magnesium concentration in the proximity of the channel pore can regulate the activity of the kinase domain [1] , [10] . In this study, we report the construction of knockout mice with the deletion of TRPM7 kinase domain. We found that although homozygous knockout mice resulted in embryonic lethality, heterozygous knockout mice were viable, but displayed abnormality in the regulation of Mg 2+ homeostasis and a defect in the intestinal Mg 2+ absorption. We also found that embryonic stem (ES) cells lacking TRPM7 kinase domain displayed a proliferation arrest phenotype that can be rescued by supplementation of extracellular Mg 2+ . Our results show that TRPM7 has an essential role in the regulation of both cellular and whole body Mg 2+ homeostasis. Deletion of TRPM7 kinase domain causes embryonic lethality To study the role of TRPM7 and its kinase domain in the regulation of Mg 2+ homeostasis in the context of the whole organism, we used a genetic approach by creating a mouse strain with a disruption of the kinase part of the TRPM7 gene. The knockout mice were obtained using a gene-targeting vector technique with further mouse colony generation ( Fig. 1a ). The gene-targeting vector was prepared using an in vivo recombination strategy. To disrupt the kinase part of TRPM7, the targeting vector was constructed for the replacement of exons 32–36 with the neomycin resistance gene cassette ( Fig. 1a ). As a result of this strategy, the TRPM7 protein is truncated immediately upstream of the alpha-kinase domain. Subsequent reverse transcription–PCR analysis of ES cells revealed that this truncation does not disrupt transcription/stability of mutant Trpm7 mRNA, which encodes a protein containing amino acids 1–1,537 of TRPM7 (see Methods section). The chimeric mice were generated and resulted in germline transmission of the Trpm7 gene with the disrupted kinase domain (TRPM7 Δ kinase ). 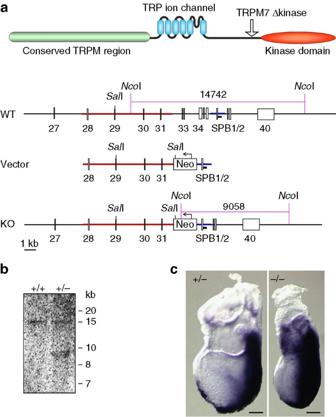Figure 1: Generation of TRPM7-deficient mice. (a) A schematic representation of TRPM7 protein. Arrow indicates the position of truncation in TRPM7Δkinasemice. Also shown are the structures of the murine TRPM7 locus, targeting vector and resulting homologous recombination locus. (b) Southern blot analysis of genomic DNA from wild-type (+/+) or TRPM7+/Δkinase(+/−) mice after digestion withNcoI. (c) TRPM7+/Δkinase(+/−) and TRPM7Δkinase/Δkinase(−/−) embryos at 7.5 days post coitum. Staining withBrachyuryantisense mRNA marks the primitive streak, where mesoderm formation occurs, and demonstrates that embryos are at the advanced primitive streak stage. Scale bar, 100 μm. Figure 1: Generation of TRPM7-deficient mice. ( a ) A schematic representation of TRPM7 protein. Arrow indicates the position of truncation in TRPM7 Δ kinase mice. Also shown are the structures of the murine TRPM7 locus, targeting vector and resulting homologous recombination locus. ( b ) Southern blot analysis of genomic DNA from wild-type (+/+) or TRPM7 +/Δ kinase (+/−) mice after digestion with Nco I. ( c ) TRPM7 +/Δ kinase (+/−) and TRPM7 Δ kinase/ Δ kinase (−/−) embryos at 7.5 days post coitum. Staining with Brachyury antisense mRNA marks the primitive streak, where mesoderm formation occurs, and demonstrates that embryos are at the advanced primitive streak stage. Scale bar, 100 μm. Full size image Out of 62 TRPM7 Δ kinase mice born from heterozygous intercrosses, none were homozygous knockout mice. Thus, knockout of TRPM7 kinase domain results in embryonic lethality. The ratio of wild type to heterozygous embryos was 22:40. It was consistent with the expected Mendelian ratio of 1:2 in the absence of knockout embryos. To determine the developmental stage at which TRPM7 kinase domain is required, we carried out timed heterozygous crossings. At 8.5 days post coitum, we observed a set of a morphologically normal embryos and a number of morphologically abnormal small necrotic embryos. All normal embryos were either heterozygous or wild type. At 7.5 days post coitum, we found TRPM7 Δ kinase/ Δ kinase embryos that were smaller in comparison with the TRPM7 +/Δ kinase or wild-type embryos. These embryos were at the advanced primitive streak stage ( Fig. 1c ). TRPM7 Δ kinase null embryos initiated gastrulation and mesoderm formation, as assessed by normal Brachyury staining ( Fig. 1c ). Thus, TRPM7 Δ kinase null embryos proceeded through a full day of gastrulation before their arrest. The early embryonic lethality of TRPM7 Δ kinase null embryos suggests that the intact kinase domain of TRPM7 is necessary for normal mouse embryonic development. In contrast to homozygous knockout mice, heterozygous TRPM7 +/Δ kinase mice were viable, which allowed for the analysis of the phenotype of these mice. TRPM7 +/Δ kinase mice exhibit altered magnesium homeostasis As TRPM7 was implicated in the regulation of magnesium homeostasis, we analysed the magnesium status of TRPM7 +/Δ kinase mice. In initial experiments, we used 8- to 9-month-old mice maintained on PicoLab Mouse Diet 20 containing 0.17% Mg 2+ . We found that, in comparison with the wild-type mice, TRPM7 +/Δ kinase mice had a significantly lower Mg 2+ concentration in plasma, urine and bones ( Table 1 ). These results demonstrate that heterozygous TRPM7 +/Δ kinase mice have altered Mg 2+ regulation. Furthermore, the response to the Mg 2+ -deficient diet was evaluated in the heterozygous TRPM7 kinase-deficient mice. The subsequent experiments were performed with 4-month-old mice maintained on semipurified diets described in the Methods section. TRPM7 +/Δ kinase mice and wild-type mice were placed on control and Mg 2+ -deficient diets with 0.1 and 0.003% Mg 2+ , respectively. They were fed these diets for 14 days before taking blood and bone samples. 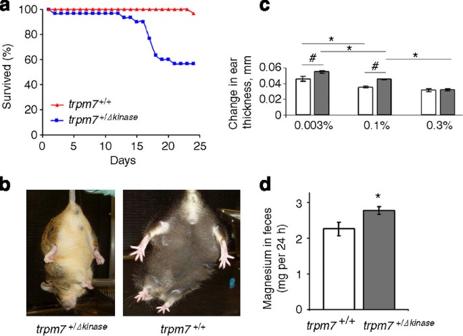Figure 2: Analysis of hypomagnesaemic phenotype in TRPM7+/Δkinasemice. (a) Survival of wild-type (TRPM7+/+) mice (n=30) or TRPM7+/Δkinasemice (n=30) on Mg2+-deficient diet. (b) Clasping test for the wild-type and TRPM7+/Δkinasemice subjected to Mg2+-free diet for 12 days. (c) The effect of TRPM7 deficiency and Mg2+content in the diet on the oxazolone sensitivity reaction. The delayed sensitivity response is measured as a change in the ear thickness, mm. Before ear application of oxazolone, wild-type mice and TRPM7+/Δkinasemice were fed for 7 days severely Mg2+deficient, control and supplemental Mg2+diet with 0.003, 0.1 and 0.3% Mg2+, respectively. The swelling response was measured 24 h after the challenge using an engineer's micrometre. Calculations of the swelling response were carried out comparing with the respective control groups not exposed to oxazolone. All mice were 4 months old. Open and shaded bars correspond to wild-type mice and TRPM7+/Δkinasemice respectively. Values are means ± s.e.m. Two-way analysis of variance test was used for the calculations (n=7–10 mice per group);P<0.05.#Significantly different from wild-type mice fed a respective diet. *Significantly different from respective wild-type or TRPM7+/Δkinasemice fed a control 0.1% Mg diet. (d) Analysis of Mg2+content in feces of the wild type mice (n=6) and TRPM7+/Δkinasemice (n=6). Mice were maintained on normal diet (0.1% Mg2+). Values are means ± s.e.m. Statistical analysis was performed by Student'st-test. *Significantly different (P<0.05). The results of these experiments revealed that with normal diet both groups of mice had no alterations in plasma or erythrocyte Mg 2+ concentration ( Table 2 ). However, the TRPM7 +/Δ kinase mice had lower levels of Mg 2+ in bones. When subjected to the Mg 2+ -deficient diet for 14 days, TRPM7 +/Δ kinase mice developed a greater decrease of Mg 2+ concentration in plasma, erythrocytes and bones than the wild-type mice ( Table 2 ). Table 1 Mg 2+ concentration in wild-type and TRPM7 +/Δkinase male mice fed PicoLab Mouse Diet 20. Full size table Table 2 Mg 2+ concentration in wild type and TRPM7 +/Δkinase mice fed diets with different Mg 2+ concentrations. Full size table We also observed a significant increase in mortality in TRPM7 +/Δ kinase mice, but not in wild-type mice placed on Mg 2+ -deficient diet ( Fig. 2a ). Also consistent with a higher sensitivity of TRPM7 +/Δ kinase mice to the low dietary Mg 2+ , after subjecting mice to 12 days of the Mg 2+ -deficient diet, we observed severe clasping of the limbs in 6 out of 10 TRPM7 +/Δ kinase mice ( Fig. 2b ). Among these six mice, three mice experienced seizures, and two mice exhibited tremor, slow movement in the cage and violent sudden leaps as a reaction to the light and noise. Clasping, tremor or seizures were never observed in 11 control wild-type mice placed on Mg 2+ -deficient diet for the same period of time. The early appearance of seizures and clasping in TRPM7 +/Δ kinase mice on Mg 2+ -deficient diet suggests the faster development of hypomagnesaemic conditions in comparison with the wild-type mice. Figure 2: Analysis of hypomagnesaemic phenotype in TRPM7 +/Δ kinase mice. ( a ) Survival of wild-type (TRPM7+/+) mice ( n =30) or TRPM7 +/Δ kinase mice ( n =30) on Mg 2+ -deficient diet. ( b ) Clasping test for the wild-type and TRPM7 +/Δ kinase mice subjected to Mg 2+ -free diet for 12 days. ( c ) The effect of TRPM7 deficiency and Mg 2+ content in the diet on the oxazolone sensitivity reaction. The delayed sensitivity response is measured as a change in the ear thickness, mm. Before ear application of oxazolone, wild-type mice and TRPM7 +/Δ kinase mice were fed for 7 days severely Mg 2+ deficient, control and supplemental Mg 2+ diet with 0.003, 0.1 and 0.3% Mg 2+ , respectively. The swelling response was measured 24 h after the challenge using an engineer's micrometre. Calculations of the swelling response were carried out comparing with the respective control groups not exposed to oxazolone. All mice were 4 months old. Open and shaded bars correspond to wild-type mice and TRPM7 +/Δ kinase mice respectively. Values are means ± s.e.m. Two-way analysis of variance test was used for the calculations ( n =7–10 mice per group); P <0.05. # Significantly different from wild-type mice fed a respective diet. *Significantly different from respective wild-type or TRPM7 +/Δ kinase mice fed a control 0.1% Mg diet. ( d ) Analysis of Mg 2+ content in feces of the wild type mice ( n =6) and TRPM7 +/Δ kinase mice ( n =6). Mice were maintained on normal diet (0.1% Mg 2+ ). Values are means ± s.e.m. Statistical analysis was performed by Student's t -test. *Significantly different ( P <0.05). Full size image Thus, under two different control diet conditions (PicoLab Mouse Diet 20 or semipurified diet), the TRPM7 +/Δ kinase mice display lower Mg 2+ bone storage. The difference in the results with plasma magnesium concentration between experiments described in Tables 1 and 2 is most likely related to the difference in mouse age and/or diet. Together with the observed higher sensitivity of the TRPM7 +/Δ kinase mice to severe dietary magnesium deficiency, particularly lower plasma and erythrocyte Mg 2+ concentrations, lower magnesium storage in the bones and cases of seizures and clasping of the limbs, the phenotype of the TRPM7 +/Δ kinase mice suggests that they have altered magnesium homeostasis. It is known that low magnesium status conditions correlate with cell-extrinsic enhancement of systemic inflammatory and allergic responses [11] . Therefore, we performed oxazolone sensitization experiments to evaluate the level of delayed-type hypersensitivity responses in TRPM7 +/Δ kinase mice. One week before sensitization, wild-type and TRPM7 +/Δ kinase mice were adapted to the control (0.1% Mg 2+ ) diet. TRPM7 +/Δ kinase mice placed on control diet, displayed an elevated oxazolone treatment sensitivity response, compared with wild-type animals ( Fig. 2c ). When wild-type and TRPM7 +/Δ kinase mice were placed on Mg-deficient diet, the hypersensitivity response was increased to a similar degree in both groups of animals ( Fig. 2c ). However, the placement of TRPM7 +/Δ kinase mice on the Mg 2+ -supplemented diet completely abrogated their hypersensitivity to oxazolone treatment, and both groups of mice displayed slightly lower responses compared with animals kept on the control diet ( Fig. 2c ). Therefore, the supplemental Mg 2+ in the diet can lower the hypersensitivity reaction of the Mg 2+ -deficient TRPM7 +/Δ kinase mice, consistent with the TRPM7 +/Δ kinase phenotype reflecting a sequelae of systemic low magnesium status as opposed to alterations in cellular physiology because of deficient TRPM7 function. Low magnesium status can arise from decreased intestinal Mg 2+ absorption, increased renal secretion or a combination of the two. Although renal excretion of Mg 2+ in TRPM7 +/Δ kinase mice was decreased (see Table 1 ), it cannot be easily determined whether this reflects a normal compensatory physiological response to preserve Mg 2+ during hypomagnesaemia or represents an inadequate compensation because of reduced TRPM7 function in our TRPM7 +/Δ kinase model. However, the effect of TRPM7 deficiency on intestinal Mg 2+ absorption can be easily and quantitatively assessed by analysing Mg 2+ content in feces from TRPM7 +/Δ kinase mice kept on a normal diet. As can be seen in Figure 2d , there was significantly higher Mg 2+ excretion in feces in TRPM7 +/Δ kinase mice in comparison with the wild-type mice (increase of 22.7%, P =0.0381), indicating that TRPM7 deficiency results in decreased intestinal Mg 2+ absorption. Deletion of the kinase domain alters TRPM7 channel properties Although we disrupted the kinase encoding part of TRPM7 gene, it is possible that this disruption affects channel function, as it was shown that the absence of the kinase domain affects TRPM7 channel sensitivity to Mg 2+ inhibition [1] , [12] . To investigate TRPM7 channel activity in TRPM7 +/Δ kinase mice, we measured TRPM7 currents in peritoneal mast cells derived from mutant and wild-type mice ( Fig. 3 ). We determined the relative expression levels of functional TRPM7 channels in the plasma membrane by recording whole-cell TRPM7-like MagNuM (magnesium nucleotide metal) currents [3] of mast cells derived from wild-type and TRPM7-deficient mice. Cells were perfused with an intracellular solution supplemented with chelators for Ca 2+ and Mg 2+ and superfused with divalent-free (DVF) external solution after full development of MagNuM ( Fig. 3a ). Under these conditions, MagNuM currents linearized to a similar degree in both genotypes as described previously for heterologously expressed TRPM7 (ref. 1 ). Currents assessed at −80 and +80 mV showed that both genotypes had similar MagNuM current amplitudes during DVF conditions, indicating that the degree of channel expression in the plasma membrane was not significantly altered. However, currents measured in cells from TRPM7 +/Δ kinase mutant mice were slightly suppressed at positive potentials ( Fig. 3b ) compared with wild-type mice. The current ratio calculated at +80 and −80 mV during DVF conditions was 0.72 for wild-type and 0.66 for TRPM7 +/Δ kinase mice. This slight suppression between wild type and TRPM7 +/Δ kinase was not caused by a change in selectivity, as the reversal potential was not significantly different in the two genotypes (wild type −7.6±1.2 mV; TRPM7 +/Δ kinase −4.9±1.2 mV, P <0.15) ( Fig. 3b ). 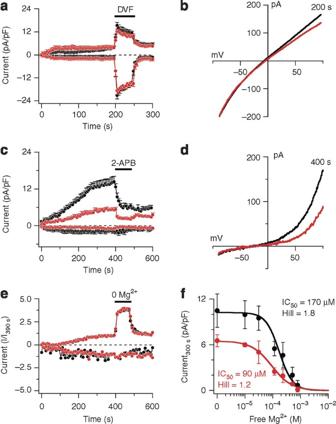Figure 3: TRPM7 (MagNuM) currents in mast cells derived from TRPM7-deficient mice. (a) Average normalized time course of MagNuM current development in mouse mast cells isolated from wild-type (black circles,n=15) and TRPM7+/Δkinasemice (red circles,n=11). Currents were elicited by a ramp protocol from −100 to +100 mV over 50 ms acquired at 0.5 Hz. Inward current amplitudes were extracted at −80 mV, outward currents at +80 mV and plotted versus time of the experiment. Data were normalized to cell size as pA/pF. Error bars indicate s.e.m. The composition of extracellular, intracellular and application solutions are described in Methods section. (b) Average current–voltage (I/V) curves extracted from a representative wild-type cell (black) and TRPM7+/Δkinase(red) extracted at 200 s. (c) Average normalized time course of MagNuM current development in mouse mast cells isolated from wild-type (black circles,n=10) and TRPM7+/Δkinasemice (red circles,n=12). Data were acquired and analysed as ina. At the time indicated by the black bar, cells were superfused with external solution supplemented with 50 μM 2-APB. (d) Current–voltage (I/V) curves extracted from a representative wild-type cell (black) and TRPM7+/Δkinase(red). (e) Average normalized time course of MagNuM current development in mouse mast cells isolated from wild-type (black circles,n=14) and TRPM7+/Δkinasemice (red circles,n=9). Data were acquired as inaand normalized as I/I390 s. Experimental solutions as ina, except for the application solution that contained (in mM) 150 NaCl, 2.8 KCl, 3 CaCl2, 10 HEPES–NaOH. Extracellular solution was nominally Mg2+free, and applied for the time indicated by the black bar. Internal solution contained 10 mM Cs-BAPTA instead of Cs-EGTA. (f) Dose–response curve of MagNuM currents to intracellular Mg2+measured in mouse mast cells isolated from wild-type (black circles,n=5–11) or TRPM7+/Δkinasemice (red circles,n=5–10). Error bars indicate s.e.m. Current amplitudes assessed at +80 mV and extracted at 300 s into the experiment. Intracellular Mg was (in μM) 0 (nominally free), 40 (31 free), 150 (116 free), 300 (233 free), 650 (507 free), 1,000 (781 free), and was calculated using WebMAXC. Figure 3: TRPM7 (MagNuM) currents in mast cells derived from TRPM7-deficient mice. ( a ) Average normalized time course of MagNuM current development in mouse mast cells isolated from wild-type (black circles, n =15) and TRPM7 +/Δ kinase mice (red circles, n =11). Currents were elicited by a ramp protocol from −100 to +100 mV over 50 ms acquired at 0.5 Hz. Inward current amplitudes were extracted at −80 mV, outward currents at +80 mV and plotted versus time of the experiment. Data were normalized to cell size as pA/pF. Error bars indicate s.e.m. The composition of extracellular, intracellular and application solutions are described in Methods section. ( b ) Average current–voltage (I/V) curves extracted from a representative wild-type cell (black) and TRPM7 +/Δ kinase (red) extracted at 200 s. ( c ) Average normalized time course of MagNuM current development in mouse mast cells isolated from wild-type (black circles, n =10) and TRPM7 +/Δ kinase mice (red circles, n =12). Data were acquired and analysed as in a . At the time indicated by the black bar, cells were superfused with external solution supplemented with 50 μM 2-APB. ( d ) Current–voltage (I/V) curves extracted from a representative wild-type cell (black) and TRPM7 +/Δ kinase (red). ( e ) Average normalized time course of MagNuM current development in mouse mast cells isolated from wild-type (black circles, n =14) and TRPM7 +/Δ kinase mice (red circles, n =9). Data were acquired as in a and normalized as I/I 390 s . Experimental solutions as in a , except for the application solution that contained (in mM) 150 NaCl, 2.8 KCl, 3 CaCl 2 , 10 HEPES–NaOH. Extracellular solution was nominally Mg 2+ free, and applied for the time indicated by the black bar. Internal solution contained 10 mM Cs-BAPTA instead of Cs-EGTA. ( f ) Dose–response curve of MagNuM currents to intracellular Mg 2+ measured in mouse mast cells isolated from wild-type (black circles, n =5–11) or TRPM7 +/Δ kinase mice (red circles, n =5–10). Error bars indicate s.e.m. Current amplitudes assessed at +80 mV and extracted at 300 s into the experiment. Intracellular Mg was (in μM) 0 (nominally free), 40 (31 free), 150 (116 free), 300 (233 free), 650 (507 free), 1,000 (781 free), and was calculated using WebMAXC. Full size image We next analysed the effect of 2-aminoethyl diphenylborinate (2-APB), an inhibitor of TRPM7, and found that its application reduced current amplitudes in wild-type and TRPM7 +/Δ kinase cells to a similar degree ( Fig. 3c ), indicating that the current was indeed carried by TRPM7 channels and that 2-APB sensitivity was not lost in mutant mast cells [13] . MagNuM currents of TRPM7 +/Δ kinase cells were significantly reduced, developing only half the amplitudes observed in wild-type mast cells ( Fig. 3c ). The comparison of the current/voltage (I/V) relationships illustrates the reduced current amplitudes for TRPM7 +/Δ kinase cells compared with wild type ( Fig. 3d ). As TRPM7 +/Δ kinase cells express a similar amount of TRPM7 channels in the plasma membrane as wild-type mast cells ( Fig. 3a and b ), the reduction of current magnitude in TRPM7 +/Δ kinase cells could be due to enhanced sensitivity of the channels to regulatory inhibitors, such as divalent ions, as half of TRPM7 molecules expressed in these cells are expected to lack the alpha-kinase domain. It has been shown that TRPM7 currents can be inhibited by extracellular magnesium [14] . We therefore assessed the sensitivity of MagNuM to removal of extracellular Mg 2+ . As Figure 3e demonstrates, replacing Mg 2+ with Ca 2+ enhanced the current response at positive potentials 2.5-fold for the wild-type and the mutant types of channels. Concentration–response curves of MagNuM currents for intracellular Mg 2+ in mast cells, isolated from wild-type or TRPM7 +/Δ kinase mice, show that MagNuM currents in TRPM7 +/Δ kinase mast cells were about two-fold more sensitive to the inhibition by intracellular Mg 2+ (wild type IC 50 =170 μM, Hill=1.8; TRPM7 +/Δ kinase IC 50 =90 μM, Hill=1.2; Fig. 3f ), indicating that the absence of one allele of the TRPM7 kinase is sufficient to increase the sensitivity to intracellular Mg 2+ dramatically. This is in good agreement with previous work, in which deletion of the TRPM7 kinase domain increased sensitivity of TRPM7 to inhibition by intracellular Mg 2+ (refs 1 , 12 ). Next, we decided to investigate TRPM7 Δ kinase null ES cells. We obtained ES cells from blastocysts of TRPM7 +/Δ kinase females after mating them with TRPM7 +/Δ kinase males. First, we measured the surface expression of TRPM7 in ES cells of all three obtained genotypes: wild type, heterozygous TRPM7 +/Δ kinase and homozygous TRPM7 Δ kinase/ Δ kinase . MagNuM currents observed in wild-type and heterozygous TRPM7 +/Δ kinase ES cells ( Fig. 4 ) were similar to those obtained in peritoneal mast cells ( Fig. 3 ). ES cells were perfused with an intracellular solution supplemented with chelators for Ca 2+ and Mg 2+ and superfused with DVF external solution after full development of MagNuM ( Fig. 4a ). Under these conditions, MagNuM currents linearized to a similar degree in wild-type and TRPM7 +/Δ kinase mutant cells, indicating that the level of channel expression in the plasma membrane was not significantly altered. However, in TRPM7 Δ kinase/ Δ kinase ES cells, DVF application resulted in much lower current amplitudes (5.5-fold) compared with wild type, suggesting a decreased expression of functional channels in the plasma membrane. The current ratio calculated at +80 and −80 mV during DVF conditions was 0.90 for wild type, 0.82 for TRPM7 +/Δ kinase and 1.22 for TRPM7 Δ kinase/ Δ kinase ES cells. Similar to our results obtained in mast cells, MagNuM currents for TRPM7 +/Δ kinase ES cells were significantly reduced compared with wild-type ES cells, whereas TRPM7 Δ kinase/ Δ kinase ES cells showed almost no MagNuM currents at all ( Fig. 4c ). The comparison of the I/V relationships illustrates the reduced current amplitudes for TRPM7 +/Δ kinase and TRPM7 Δ kinase/ Δ kinase cells compared with wild type ( Fig. 4d ). Thus, our electrophysiological studies of mast cells and ES cells suggest that the deletion of TRPM7 kinase domain reduces channel activity and increases its sensitivity to magnesium inhibition. 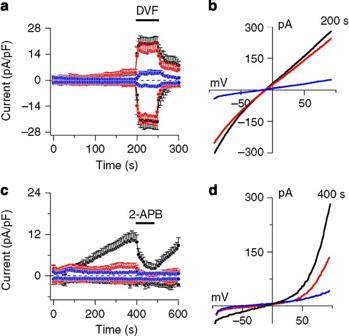Figure 4: TRPM7 (MagNuM) currents in ES cells derived from TRPM7 deficient mice. (a) Average normalized time course of TRPM7 current development in mouse ES cells isolated from wild-type (black circles,n=13), TRPM7+/Δkinase(red circles,n=12) and TRPM7Δkinase/Δkinasemice (blue circles,n=13). Data were acquired and analysed as inFigure 3a. Error bars indicate s.e.m. The intracellular solution was divalent-free and contained (in mM) 140 Cs-glutamate, 8 NaCl, 10 Cs-EGTA, 5 Na-EDTA (pH 7.2, 300 mOsm). The extracellular solution contained (in mM) 140 NaCl, 1 CaCl2, 2.8 KCl, 2 MgCl2, 10 HEPES–NaOH, 11 glucose (pH 7.2, 300 mOsm). The application solution contained (in mM) 150 mM NaCl, 2.8 KCl, 10 HEPES–NaOH, 0.5 Na-EDTA. (b) Average current–voltage (I/V) curves from a representative wild-type cell (black), TRPM7+/Δkinase(red) and TRPM7Δkinase/Δkinase(blue) extracted at 200 s. (c) Average normalized time course of MagNuM current development in mouse ES cells isolated from wild-type (black circles,n=8), TRPM7+/Δkinasemice (red circles,n=10) and TRPM7Δkinase/Δkinasemice (blue circles,n=10). Data were acquired and analysed as ina. At the time indicated by the black bar, cells were superfused with external solution supplemented with 50 μM 2-APB. (d) Current–voltage (I/V) curves extracted from a representative wild-type cell (black), TRPM7+/Δkinase(red) and TRPM7Δkinase/Δkinase(blue). Figure 4: TRPM7 (MagNuM) currents in ES cells derived from TRPM7 deficient mice. ( a ) Average normalized time course of TRPM7 current development in mouse ES cells isolated from wild-type (black circles, n =13), TRPM7 +/Δ kinase (red circles, n =12) and TRPM7 Δ kinase/ Δ kinase mice (blue circles, n =13). Data were acquired and analysed as in Figure 3a . Error bars indicate s.e.m. The intracellular solution was divalent-free and contained (in mM) 140 Cs-glutamate, 8 NaCl, 10 Cs-EGTA, 5 Na-EDTA (pH 7.2, 300 mOsm). The extracellular solution contained (in mM) 140 NaCl, 1 CaCl 2 , 2.8 KCl, 2 MgCl 2 , 10 HEPES–NaOH, 11 glucose (pH 7.2, 300 mOsm). The application solution contained (in mM) 150 mM NaCl, 2.8 KCl, 10 HEPES–NaOH, 0.5 Na-EDTA. ( b ) Average current–voltage (I/V) curves from a representative wild-type cell (black), TRPM7 +/Δ kinase (red) and TRPM7 Δ kinase/ Δ kinase (blue) extracted at 200 s. ( c ) Average normalized time course of MagNuM current development in mouse ES cells isolated from wild-type (black circles, n =8), TRPM7 +/Δ kinase mice (red circles, n =10) and TRPM7 Δ kinase/ Δ kinase mice (blue circles, n =10). Data were acquired and analysed as in a . At the time indicated by the black bar, cells were superfused with external solution supplemented with 50 μM 2-APB. ( d ) Current–voltage (I/V) curves extracted from a representative wild-type cell (black), TRPM7 +/Δ kinase (red) and TRPM7 Δ kinase/ Δ kinase (blue). Full size image Supplemental Mg 2+ rescues growth of TRPM7-deficient ES cells To test whether the growth pattern and magnesium requirements are changed in the mutant ES cells, equal amounts of wild-type, heterozygous TRPM7 +/Δ kinase and homozygous TRPM7 Δ kinase/ Δ kinase ES cells were grown in control ES-Dulbecco's modified Eagle's medium (DMEM) and ES-DMEM supplemented with 10 mM MgCl 2 . After 72 h of growth, the ES cells were observed and images were taken using phase-contrast microscopy. 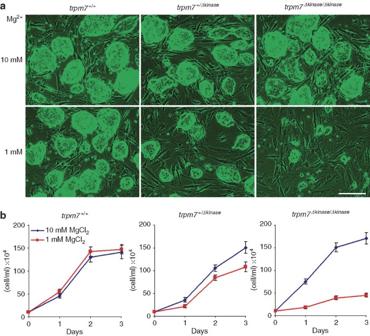Figure 5: Mg2+supplementation rescues the growth arrest phenotype of TRPM7 deficient ES cells. Equal amounts (2.2 × 105per well) of wild-type, TRPM7+/Δkinaseand TRPM7Δkinase/ΔkinaseES cells were plated in six-well plates in 2 ml of the control ES-DMEM and ES-DMEM supplemented with 10 mM MgCl2. (a) Phase-contrast images were taken after 72 h of growth. Scale bar, 200 μm. (b) Growth curves. Number of ES cells were quantified at different time points. Error bars indicate s.e.m.,n=3. As Figure 5 demonstrates, at 72 h after plating, ES homozygous TRPM7 Δ kinase/ Δ kinase cells did not grow significantly in the control media containing 1 mM MgCl 2 . However, supplementation with 10 mM MgCl 2 rescued the growth inhibition phenotype of TRPM7 Δ kinase/ Δ kinase ES cells. TRPM7 Δ kinase/ Δ kinase ES cells grown in 10 mM MgCl 2 appeared as healthy and confluent as wild-type ES cells grown in 1 mM MgCl 2 control media for 72 h. When the concentration of MgCl 2 in the media was increased from 1 mM to 10 mM, the ES TRPM7 Δ kinase/ Δ kinase cell growth fully recovered and confluence was reached in 48 h. The heterozygous ES cells presented an intermediate growth inhibition effect in media containing 1 mM MgCl 2 . These results suggest that TRPM7 has an essential role in the proliferation of ES cells probably by providing the necessary Mg 2+ influx. Interestingly, we found that ES cells express TRPM6 mRNA and its level was similar in wild-type and TRPM7 Δ kinase/ Δ kinase cells ( Supplementary Fig. S1 ). These results suggest that TRPM6 cannot compensate the deficiency of TRPM7 in ES cells. Figure 5: Mg 2+ supplementation rescues the growth arrest phenotype of TRPM7 deficient ES cells. Equal amounts (2.2 × 10 5 per well) of wild-type, TRPM7 +/Δ kinase and TRPM7 Δ kinase/ Δ kinase ES cells were plated in six-well plates in 2 ml of the control ES-DMEM and ES-DMEM supplemented with 10 mM MgCl 2 . ( a ) Phase-contrast images were taken after 72 h of growth. Scale bar, 200 μm. ( b ) Growth curves. Number of ES cells were quantified at different time points. Error bars indicate s.e.m., n =3. Full size image Our results that TRPM7 deficiency in ES cells leads to the inhibition of proliferation are consistent with previous reports, showing that deletion of TRPM7 in DT-40 cells arrests cell cycle progression. It was demonstrated that at standard magnesium concentration TRPM7-deficient DT-40 cells become arrested in a quiescent G0-like state [15] . They can be induced to progress through cell cycle by increasing extracellular magnesium concentration [1] or by overexpressing SLC41A2 magnesium transporter [16] . What can be the role of TRPM7 in cell proliferation? Free magnesium represents only 1–2% of total intracellular magnesium [17] and most intracellular magnesium is bound to ATP, other nucleotide phosphates, RNA, proteins and membranes. As most cell constituents are doubled in their amount during G1 phase of the cell cycle, it is expected that a large amount of additional magnesium is needed to bind newly synthesized molecules. This explains why reduction of extracellular magnesium inhibits cell proliferation [18] , [19] , [20] and why magnesium is required specifically during G1 phase of the cell cycle [18] . Interestingly, it was shown that TRPM7 current is kept at a low level at G0, S, G2 and M phases of the cell cycle and becomes activated specifically during G1 phase [21] . Therefore, it is likely that TRPM7 mediates magnesium influx during G1 phase of the cell cycle and this represents its primary function in the regulation of cellular magnesium homeostasis. In addition to its role in the regulation of cellular magnesium homeostasis in proliferating cells, our results suggest that TRPM7 also has a key role in the regulation of whole body Mg 2+ balance. It has been previously proposed that another channel kinase TRPM6 regulates Mg 2+ homeostasis at the level of the organism [1] , [4] , [5] . Indeed, only mutations in TRPM6 but not TRPM7 have been reported in patients with hypomagnesaemia. However, observations by Chubanov et al . [22] , [23] subsequently suggested a refined model, in which TRPM6 exerts its action on Mg 2+ absorption through heteromultimeric channels formed in association with TRPM7, as TRPM6 was found to be unable to assemble functional channels unless coexpressed with TRPM7 (refs 22 , 23 ). Our results would be consistent with this refined model, as we observe a defect in intestinal Mg 2+ absorption in TRPM7 +/Δ kinase mice, reminiscent of that observed in TRPM6-deficient patients, although we cannot exclude an additional deficit in Mg 2+ uptake through dysregulated TRPM7 homomultimeric channels as well. Interestingly, magnesium urinary excretion values are significantly lower in TRPM7 +/Δ kinase mice (see Table 1 ), suggesting that either deletion of the kinase domain does not negatively affect TRPM7 +/Δ kinase function in the kidney or that TRPM7 +/Δ kinase mice activate some compensatory mechanisms that help increase magnesium reabsorbtion in the kidney. Recently, Walder et al . [24] demonstrated that TRPM6 +/- mice had lower plasma Mg 2+ levels, but no difference in urinary or fecal Mg 2+ concentrations compared with wild-type mice. In comparison, TRPM7 +/Δ kinase mice had a significant increase in Mg 2+ excretion in feces suggesting that TRPM7 deficiency in mice has a stronger effect on intestinal Mg 2+ absorption than TRPM6 deficiency. Taken together, our results indicate that (1) impaired function of TRPM7 conductance results in dysregulation of Mg 2+ homeostasis in mammalian organisms; (2) TRPM6 cannot compensate for the decrease in TRPM7 channel or the loss of TRPM7 kinase function, but conversely TRPM7 may interfere with functional TRPM6 channels by forming heteromultimeric channels; (3) the loss of the TRPM7 kinase domain might trigger further yet unknown mechanisms, culminating in a low magnesium, hyperallergic phenotype. Our results are consistent with the following model of TRPM7 functioning. At the cellular level, TRPM7 may serve as an Mg 2+ channel, in which activity is regulated by intracellular Mg 2+ through a negative feedback mechanism. TRPM7 is particularly important to ensure a rapid Mg 2+ entry during G1 phase of the cell cycle. Therefore, deficiency of TRPM7 in DT-40 cells or ES cells results in the arrest of cell proliferation because of the inability to traverse the G1 phase of the cell cycle. Our results suggest that TRPM7 is also involved in whole body Mg 2+ homeostasis. Whole body Mg 2+ influx is provided by Mg 2+ absorption in the intestine and reabsorbtion in the kidney. We found that TRPM7 is essential for normal Mg 2+ absorption in the intestine. This suggests that in cells mediating transcellular magnesium transport TRPM7 is active even in non-proliferating cells. Therefore, there should be additional mechanisms that activate TRPM7 in tissues with transcellular Mg 2+ transport. As TRPM6 is expressed predominantly in the intestine and kidney and can form heteromeric complexes with and activate TRPM7 (ref. 22 ), it is tempting to suggest that the primary function of TRPM6 may be to enhance the function of TRPM7 in tissues with transcellular magnesium transport. In addition, the expression of TRPM6 in ES cells (see Supplementary Fig. S1 ) and during early embryonic development [24] may be related to the requirement of rapidly dividing cells of the embryo for high amounts of Mg 2+ . Taken together, our data show that TRPM7 is essential for embryonic development and systemic Mg 2+ homeostasis in a mammalian organism. The latter result is in contrast to a recent study [25] , in which a targeted deletion of TRPM7 in mouse thymic medullary cells reportedly did not alter acute uptake of Mg 2+ or maintenance of total cellular Mg 2+ . It was therefore concluded that TRPM7 is not essential for cellular Mg 2+ homeostasis in mice. One of the possible explanations of this discrepancy between their conclusions and ours is that Jin et al . [25] analysed cells in a quiescent state, in which TRPM7 may not be important for the regulation of magnesium influx. Also the experimental approaches presented by Jin et al . [25] are not clear-cut and may not be suitable to exclude Mg 2+ regulation as the critical defect. First, Mg 2+ influx was studied using the fluorescent indicator KMG104AM, and Mg 2+ influx was evaluated in the absence and presence of high extracellular Mg 2+ in T lymphocytes isolated from wild-type and TRPM7 -/fl (lck-Cre) mice. Although intracellular Mg 2+ increased during extracellular exposure to 10 mM Mg 2+ , no difference in fluorescent signal, and therefore Mg 2+ influx, was found between wild-type and mutant cells. However, this is not an unexpected result, as it is not related to TRPM7 activity. Mg 2+ entering the cell through TRPM7 during high extracellular Mg 2+ conditions will exert negative feedback inhibition on TRPM7 channels, thus shutting down channel activity and in turn suppress Mg 2+ influx within a few seconds [6] . Hence, the absence or presence of TRPM7 channels in mutant or wild-type T cells is irrelevant under high external Mg 2+ conditions, and any increase in cellular Mg 2+ simply reflects Mg 2+ influx through pathways independent of TRPM7. Therefore, a further pharmacological suppression by 2-APB is also not expected to have any additional effects on Mg 2+ influx. The third experimental approach chosen by Jin et al . [25] assessed differences in Mg 2+ influx in thymocytes isolated from wild-type and TRPM7 -/fl (lck-Cre) mice during extracellular acidification, which causes a strong potentiation of inward currents compared with outward currents assessed at −80 and +80 mV, respectively. However, this increase in inward ion flux does not translate into an increased Mg 2+ flux, as acidification causes a change in ion selectivity favouring monovalent over divalent ions. Importantly, decreases in extracellular pH do not affect divalent cation conductance [26] . Therefore, extracellular acidification experiments are not suited to assess changes in Mg 2+ influx through TRPM7 channels. Finally, the inability to detect differences in total cellular Mg 2+ between wild-type and TRPM7 -/fl (lck-Cre) T cells could indicate that steady-state levels of cellular Mg 2+ are not compromised and that these cells, given enough time, have mechanisms to regulate cellular Mg 2+ homeostasis, despite deficiencies in acute Mg 2+ influx, especially in light of the fact that the systemic Mg 2+ homeostasis and Mg 2+ plasma levels are not affected in TRPM7 -/fl (lck-Cre) mice. The incomplete knock-out of TRPM7, in which reportedly a significant portion of T cells maintain TRPM7 expression [25] , would also allow for some regulation of Mg 2+ contents by TRPM7 in a subset of tested cells. In contrast, our use of a uniformly expressed TRPM7 hypomorphic allele allowed us to manipulate and analyse murine Mg 2+ physiology at the whole animal level, and we observe clear effects on systemic Mg 2+ homeostasis in association with deficient TRPM7 function. Overall, our findings with mice genetically deficient in TRPM7 function represent the first direct evidence, implicating TRPM7 in the control of whole body Mg 2+ levels, and place TRPM7 at the nexus of mechanisms that regulate both cellular and whole body Mg 2+ homeostasis. Construction of TRPM7 Δ kinase mice All animal procedures were approved by the Institutional Animal Care and Use Committee (IACUC) and adhered to principles outlined in the National Institutes of Health Guide for the Care and Use of Laboratory Animals. Experiments in A. Mazur laboratory were performed according to the guidelines of the INRA Ethics Committee, in accordance with decree no. 87–848. The knockout mice were obtained using a gene-targeting vector technique for TRPM7 with further mice colony generation. The gene-targeting vector was prepared using an in vivo recombination strategy. To disrupt the kinase domain of the TRPM7, the targeting vector was constructed by using a short arm 1.3 kb DNA fragment of an intron located between exons 36 and 37. The short arm was a PCR fragment from AKASA2 to AKASA1. AKASA2 is located 222 bp downstream of exon 36, with a sequence of 5′-GTAACTTTCCTGCCCGAGTCTC-3′. AKASA1 is located 116 bp upstream of exon 37 with a sequence of 5′-CTTATCTCTCAAGCCAATTTAGGAG-3′. The short arm was inserted into the 5′ of the Neo gene cassette using Mlu I site. The long arm was a 9.7 kb genomic fragment containing exons 28–31. In this strategy, exons 32–36 encoding the large portion of the kinase domain were replaced by the Neo gene cassette ( Fig. 1 ). As a result, the TRPM7 protein is truncated immediately upstream of the alpha-kinase domain. The reverse transcription–PCR analysis of ES knockout cells (see Supplementary Fig. S2 ) showed that TRPM7Δkinase protein contains TRPM7 amino acids 1–1,537 and an additional stretch of 48 amino acids with the following sequence: DLQRIDPLRRTRQEGDRRRCAANRERRYRKARGSGQPIRRQALQQYHG. The targeting vector was linearized by Not I and then transfected by electroporation into 129 SV ES cells. After selection with G418, surviving colonies were expanded, and PCR analysis was performed to identify clones that had undergone homologous recombination. The correctly targeted ES cell lines were microinjected into C57BL/6J blastocysts. The chimeric mice were generated and resulted in germline transmission of the trpm7 gene with the disrupted kinase domain. The knockout of one allele in heterozygous TRPM7 +/Δkinase mice was confirmed by Southern blot analysis ( Fig. 1b ). Preparation of ES cells for construction of TRPM7 Δkinase mice and implantation were performed at inGenious Targeting Laboratory, Stony Brook, NY. Isolation of the peritoneal mast cells and primary cell culture Cells were isolated from the peritoneum of wild-type or TRPM7 +/Δ kinase mice, collected in standard external saline through lavage of the abdomen, and centrifuged at 1,000 r.p.m. for 10 min. The pellet was resuspended in 1 ml DMEM and placed into two Petri dishes with up to five poly-d-lysine-coated glass coverslips. Cells were cultured in 2 ml DMEM containing 10% fetal bovine serum and 1% Penicillin/Streptomycin overnight and subsequently used for experiments up to the second day after isolation. Mast cells were identified visually using light microscopy (phase contrast) according to their distinct dark appearance and their characteristic nucleus. Electrophysiology Patch-clamp experiments were performed in the tight-seal whole-cell configuration. High-resolution currents were acquired and recorded using EPC-9 (HEKA) and PatchMaster (HEKA). All voltages were corrected for a liquid junction potential of 10 mV between external and internal solutions. Currents were elicited by a ramp protocol from −100 to +100 mV over 50 ms acquired at 0.5 Hz and a holding potential of 0 mV. Inward current amplitudes were extracted at −80 mV, outward currents at +80 mV, normalized to cell size and plotted versus time of the experiment. Standard extracellular solution contained (in mM) 140 NaCl, 1 CaCl 2 , 2.8 KCl, 2 MgCl 2 , 10 HEPES–NaOH, 11 glucose (pH 7.2, 300 mOsm). DVF intracellular solution contained (in mM) 140 Cs-glutamate, 8 NaCl, 10 Cs-EGTA, 5 Na-EDTA (pH 7.2, 300 mOsm). The extracellular Mg 2+ -free application solution contained (in mM) 150 NaCl, 2.8 KCl, 3 CaCl 2 , 10 HEPES–NaOH (pH 7.2, 300 mOsm). For Mg 2+ dose–response experiments, the current amplitudes were assessed from ramp currents at +80 mV obtained 300 s into the experiment. Nominally, Mg 2+ -free extracellular solution for the MgCl 2 dose–response experiments contained 3 mM CaCl 2 to substitute for the loss of divalents (in mM): 150 NaCl, 3 CaCl 2 , 2.8 KCl, 0 MgCl 2 , 10 HEPES–NaOH, 11 glucose (pH 7.2, 300 mOsm); intracellular solution contained (in mM) 140 Cs-glutamate, 8 NaCl, 10 Cs-BAPTA plus appropriate amount of MgCl 2 was added, as calculated with WebMaxC. Mg 2+ measurements in murine biological samples The 4-month-old wild-type and TRPM7 +/Δ kinase male mice were fed the control (0.1% Mg 2+ ), severely Mg 2+ -deficient (0.003% Mg 2+ ) or Mg 2+ -supplemented (0.3%) diet for the appropriate period of the experiments. The magnesium concentrations in the experimental diets were determined by flame atomic absorption spectrophotometry (Perkin Elmer 800) at 285 nm. All mice had free access to distilled water and food. The semipurified diets contained the following (g kg −1 ): casein 200, starch 650, corn oil 50, alphacel (cellulose) 50, DL-methionine 3, choline bitartrate 2, modified AIN-76 mineral mix 35, AIN-76A vitamin mix 10 (ICN Biomedicals). MgO was omitted from the mineral mix in magnesium-deficient diet. At the end of the experimental period, mice were anaesthetized with sodium pentobarbital (40 mg kg −1 per body weight). Blood was obtained by puncturing the abdominal vein with a heparinized syringe. Blood samples were centrifuged at 1,000 g for 10 min at 20 °C, and the plasma and erythrocytes were then stored at −20 °C. Before killing the mice, 24-h urine sample was collected in metabolic cages and acidified with HCl (final pH <2). For total magnesium determination, plasma, haemolysed erythrocytes and urine were diluted in 0.1% lanthanum chloride. For bones and feces, the samples were weighed, dry-ashed (10 h at 500 °C) and dissolved with concentrated HNO 3 (14 M) and H 2 O 2 (30%), on a heating plate until complete discoloration was achieved. The mineral solution was adjusted to 10 ml with distilled water and diluted with 0.1% lanthanum chloride as previously described [27] , [28] . The Mg 2+ content was determined by atomic absorption spectrophotometry (Perkin Elmer AA800) at 28.5. Isolation and culture of mouse ES cells Isolation and culture of blastocyst-derived stem cells were carried out according to the protocols described in the laboratory manual for manipulating the mouse embryo [29] . The media used for isolation and culture of ES cells was supplemented with 10 mM MgCl 2 . Primary cultures of mouse embryonic fibroblasts were used as feeder cells. To prepare mitotically inactive feeder cells, mouse embryonic fibroblasts were treated with Mitomycin C (Sigma). Images of ES cells were obtained with a phase-contrast ×10 UplanFI objective using an Olympus IX70 microscope equipped with an environmental chamber at a temperature of 37 °C. Cell counting was performed using a hemocytometer. Southern blotting For Southern blot analysis, genomic DNA (10 μg) was digested with Nco I at 37 °C for 5 h. Digested DNA was loaded on 0.8% agarose gel and fractionated by electrophoresis. After denaturing and neutralizing, DNA was transferred onto nylon membrane and crosslinked by ultraviolet light. The membrane was prehybridized at 42 °C for 4 h. 32 P-labelled probe was then added and hybridization was performed at 42 °C overnight. The signal was detected by a phosphorimager. Embryo collection and whole-mount in situ hybridizations Whole-mount in situ hybridizations were performed as previously described [30] . DNA template was generated from mouse cDNA encoding Brachyury. The antisense RNA probe was synthesized from 1 μg of linearized cDNA and labelled with digoxigenin-UTP (Roche) using SP6 RNA polymerase (Promega). The transcription reaction was carried out at 37 °C for 2 h, followed by DNaseI treatment (Promega). Embryos were dissected and fixed overnight in 4% paraformaldehyde (PFA) in phosphate-buffered saline (PBS) at 4 °C. After an overnight fixation tissues were washed in PBS containing 0.1% Tween-20 (PBT). Following dehydration, the tissues were stored in 100% methanol at −20 °C until use. After rehydration in PBT, embryos were bleached in 6% peroxide solution for 1 h, permeabilized with proteinase K (10 mg ml −1 ) for 1 min, and postfixed in 4% PFA plus 0.2% glutaraldehyde. Proteinase K was inactivated with 0.2% glycine in PBT. Samples were incubated in hybridization buffer (50% formamide) for 2 h at 70 °C and then hybridized at the same temperature with 0.5 μg ml −1 labelled RNA probe overnight. After posthybridization washes and RNase-A treatment (100 μg ml −1 ), tissues were rinsed 3×5 min in maleic acid buffer (MAB; 0.1 M maleic acid, pH 7.5, 0.15 M NaCl, 0.1% Tween-20 and 0.002 M levamisole) and then incubated in blocking buffer (MAB+10% sheep serum, and 2% blocking reagent (Roche)), at room temperature for 3 h. Hybridized probes were incubated with preabsorbed anti-digoxigenin-AP (Roche) diluted 1:4,000 in blocking buffer (Roche) containing 3 mg of mouse embryo powder overnight at 4 °C. Embryos were washed several times with MAB over a 24-h period at room temperature, and then developed with BM purple (Roche) colour substrate for 5–16 h. Reactions were then stopped with 3×5 min PBT, postfixed in 4% PFA plus 0.2% glutaraldehyde, and stored in 80% glycerol in PBT. Embryos were dissected and viewed on a LeicaMZ7 5 stereoscope. Embryos were photographed in 80% glycerol with a LeicaMZFLII stereoscope equipped with a Zeiss Axiocam HR digital camera, and Zeiss Axiovision version 4.5 imaging software. Clasping test Hindlimb clasping test was performed on day 12 of the Mg-deficient diet for both TRPM7-deficient and wild-type control mice. The clasping test evaluated the mice hindlimb response during suspension by the tail 10 cm above their home cage. Each mouse was observed during the first 5 s of suspension and evaluated as having normal or abnormal movement and positioning of the limbs. When the mouse held its hindlimbs outward to steady itself, its hindlimb movements were considered normal and the mouse was defined as clasping negative. When the mouse made dystonic movement of the hindlimbs with clasping, where the limbs were pulled close to the body axis, its hindlimb movements were considered abnormal, and the mouse was defined as clasping positive. Delayed hypersensitivity response measurements Oxazolone was used as a contact-sensitizing agent. Oxazolone (0.5%) dissolved in acetone was applied on the shared mouse abdomen immediately before placing mice on experimental diets with various Mg 2+ content. Control animals were exposed to vehicle alone. Six days after sensitization, mice were challenged by epicutaneous application of 1% oxazolone in acetone on the ears. The swelling response was measured 24 h after challenge using an engineer's micrometer. Calculations of the swelling response were carried out by comparing to the respective control groups not exposed to oxazolone. How to cite this article: Ryazanova, L. V. et al . TRPM7 is essential for Mg 2+ homeostasis in mammals. Nat. Commun. 1:109 doi: 10.1038/ncomms1108 (2010).